Electronic control of H+current in a bioprotonic device with Gramicidin A and Alamethicin In biological systems, intercellular communication is mediated by membrane proteins and ion channels that regulate traffic of ions and small molecules across cell membranes. A bioelectronic device with ion channels that control ionic flow across a supported lipid bilayer (SLB) should therefore be ideal for interfacing with biological systems. Here, we demonstrate a biotic–abiotic bioprotonic device with Pd contacts that regulates proton (H + ) flow across an SLB incorporating the ion channels Gramicidin A (gA) and Alamethicin (ALM). We model the device characteristics using the Goldman–Hodgkin–Katz (GHK) solution to the Nernst–Planck equation for transport across the membrane. We derive the permeability for an SLB integrating gA and ALM and demonstrate pH control as a function of applied voltage and membrane permeability. This work opens the door to integrating more complex H + channels at the Pd contact interface to produce responsive biotic–abiotic devices with increased functionality. From electroceuticals [1] to wearable devices [2] , and from electronic plants [3] to edible electronics [4] , interfacing electronic devices with biological systems promises new therapies and device functionalities beyond silicon [5] , [6] . In biological systems, most of the communication between cells is mediated by membrane proteins and ion channels that passively allow or actively control the flow of ions and small molecules across the cell membrane [7] . In this fashion, complex functions such as muscle contraction, neuronal signalling and metabolism are achieved. Membrane proteins are studied using patch clamps [8] , micropore arrays [9] and electrode-supported lipid bilayers [10] , [11] , [12] , [13] , and passive transmembrane ionic transport is controlled by local electrical and chemical potential gradients according to the Nernst–Planck equation [14] , [15] . While most common ions are Na + , K + and Cl − , proton (H + ) currents and concentration [ H + ] gradients play important physiological roles [16] . Examples include oxidative phosphorylation in mitochondria [17] , light-activated H + pumping by archaeal bacteriorhodopsins [18] , H + -activated bioluminescence in dinoflagellates [19] , flagellar propulsion in bacteria [20] , voltage gated H + channels [21] and antibiotic action by polypeptides such as Gramicidin [22] . Ionic currents and membrane proteins are the most intimate interface for electronics to communicate with cells and biological systems [23] . However, conventional electronics typically use electrons as charge carriers instead of ions. To address this issue, gramicidin and bacteriorhodopsin have been integrated as gating elements with carbon nanotubes [24] , silicon nanowires [25] and organic field effect transistors [26] to develop biosensors with increased functionality. Organic polymers [27] , [28] , [29] with ionic [30] , [31] and mixed conductivity have been used to record and stimulate physiological functions and even assembled into logic circuits [32] . We have recently demonstrated control of H + flow in bioprotonic field effect transistors (H + -FETs) [33] , [34] , [35] and memories [36] , and integrated these devices with enzymatic logic gates [37] . H + -FETs built with squid reflectin proteins have also been described [38] , [39] , [40] . At the heart of these devices is the use of the Pd/PdH x couple as a contact that enables the translation of an H + current into an electronic current and thus serves as a transducer between biological systems and electronics [35] , [41] . Here, we fabricate and characterize bioprotonic devices incorporating ion channels and Pd/PdH x contacts to control H + currents and modulate pH gradients across phospholipid membranes ( Fig. 1 ). These devices comprise a supported lipid bilayer (SLB) that mimics the function of a cell membrane at the Pd/solution interface and acts as a self-sealing support for the insertion of the ion channels Gramicidin A (gA) and Alamethicin (ALM). We show that gA can be used to linearly control H + currents as function of voltage while ALM functions as a voltage-gated channel analogous to an ON-OFF switch. This is a unique and novel architecture compared to prior work with electron conducting Au [42] and Pt [43] electrodes that allows for direct interfacing of H + current from the ion channels. 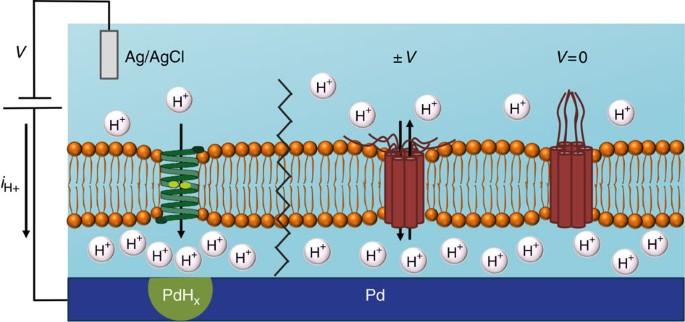Figure 1: Schematic depiction of the ion channel bioprotonic device. (Left) A bioprotonic device with integrated Gramicidin (gA) supports the flow of H+across the SLB upon application of a negative voltage (−V) to the Pd contact. When H+reach the surface of the Pd contact, they are reduced to H by an incoming electron and diffuse into Pd to form a hydride (PdHx). A reduction current at the Pd contact is measured as current density (−iH+). (Right) In a bioprotonic device with integrated Alamethicin (ALM), applying a negative or positive voltage (V) above a threshold value at the Pd contact opens the gate and allows H+flow across the SLB, turning the device ON. AtV=0 mV, no H+flows across ALM and the device switches OFF. Figure 1: Schematic depiction of the ion channel bioprotonic device. (Left) A bioprotonic device with integrated Gramicidin (gA) supports the flow of H + across the SLB upon application of a negative voltage ( −V ) to the Pd contact. When H + reach the surface of the Pd contact, they are reduced to H by an incoming electron and diffuse into Pd to form a hydride (PdH x ). A reduction current at the Pd contact is measured as current density (− i H+ ). (Right) In a bioprotonic device with integrated Alamethicin (ALM), applying a negative or positive voltage (V) above a threshold value at the Pd contact opens the gate and allows H + flow across the SLB, turning the device ON. At V =0 mV, no H + flows across ALM and the device switches OFF. Full size image Device architecture Pd contacts are evaporated in areas ranging from 10 μm 2 (2 × 5 μm) to 200 μm 2 (2 × 100 μm) onto a Si wafer with a 100 nm SiO 2 insulating layer. Microfluidic channels are defined by lithographically patterned SU-8 photoresist and sealed with a polydimethylsiloxane layer comprising of inlet and outlet ports ( Supplementary Fig. 1 ). The channels are filled with a standard buffered solution (5 mM PBS and 100 mM KCl, pH=7.0) and an Ag/AgCl electrode is inserted into the solution to serve both as a reference electrode and as a counter electrode in a two terminal setup. We apply a potential difference between the Pd contact and the Ag/AgCl electrode ( V ) and measure the resulting H/H + current density ( i H+ ) where oxidation of H corresponds to a positive i H+ and reduction of H + corresponds to a negative i H+ ( Fig. 1 ). For − V applied to the Pd contact, electrons flow from the Pd contact and reduce H + to H at the Pd/solution interface. H then absorbs into the Pd to form PdH x with x up to 0.6. Conversely, for + V , H oxidizes into H + at the Pd/solution interface, and is released into solution. This results in the collection of electrons by the Pd contact, which in turn yields a positive i H+ value. In short, by measuring i H+ , we effectively monitor the flow of H + between the solution and the Pd contact mediated by H + +e − ⇔ H, and subsequent absorption of H into Pd to form PdH x or desorption of H from the contact to form H + (refs 37 , 44 ). To electrically isolate the Pd contact from the solution and provide a template for ion channel insertion, we deposit a 1,2-Dioleoyl-sn-glycero-3-phosphocholine (DOPC, Sigma-Aldrich Lipids) SLB onto the Pd contact using vesicle fusion [45] . Force rupture measurements by Atomic Force Microscopy (AFM) [46] show that the thickness of the SLB membrane is 4.8±0.7 nm ( n =20, for a device with dimension of 2 × 50 μm), which is close to the expected value of 5.5 nm for a DOPC bilayer [47] , [48] ( Supplementary Fig. 2 and Supplementary Note 1 ). In essence, the SLB mimics a cell membrane that electrically insulates the Pd contact ( ρ ∼ 3 G Ω cm −1 ; see Supplementary Fig. 3 and Supplementary Table 1 ) and divides the solution into two volumes. We refer to the larger volume containing the Ag/AgCl electrode as the bulk solution (B). We refer the small volume between the SLB and the Pd contact, as the isolation layer (IL). The IL provides lubrication and mobility to the SLB [49] , [50] , [51] , [52] , creating an excellent platform for the investigation of cellular processes involving small size molecules such as gA and ALM. Voltage control of H + flow with Gramicidin A Gramicidin A (gA) is a short helical polypeptide from Bacillus brevis that dimerizes in lipid bilayers to form a transmembrane channel that allows the passage of small cations (including H + ) while remaining impermeable to anions [53] . To control the flow of H + as a function of V , we integrate gA in the SLB of our devices. In the absence of gA and at an applied V =−200 mV, we measure i H+ =−1.2 mA cm −2 ( Fig. 2a,d ). This small i H+ indicates that few H + diffuse across the bilayer to become reduced at the Pd surface. To confirm this result, we set V =0 mV after applying V =−200 mV for 10 min. If any H + flow were to occur across the SLB during the V =−200 mV step, a significant amount of PdH x should form at the Pd/solution interface [37] . This PdH x has a higher protochemical potential ( μ H+ ) than the solution of pH=7.0 at V =0 mV, leading to H oxidation at the PdH x contact, H + flow from the PdH x into the IL, and giving rise to a measurable positive i H+ (ref. 34 ). The black trace in Fig. 2d (right hand side panel) shows that this is clearly not the case. 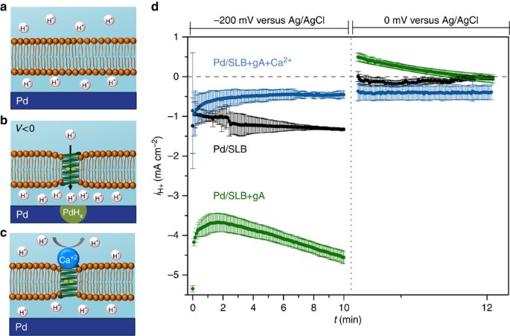Figure 2: Schematics of bioprotonic gA devices. (a) Pd contact coated with a SLB. The SLB inhibits the flux of H+from the bulk solution to the Pd/solution interface. (b) Pd contact with SLB incorporating gA is semipermeable to H+, with gA channels facilitating the rapid flow of H+to the Pd/solution interface. (c) Addition of 1 mM Ca2+to the bulk solution, blocks gA and prevents the flow of H+to the Pd/solution interface. (d)iH+versus time plot forV=−200 mV andV=0 mV. Black trace SLB, green trace SLB+gA, blue trace SLB+gA blocked by Ca2+. (The data are collected from 3 different devices with different dimensions: Pd / SLB: 3 different devices of 2 × 50 μm, Pd/SLB+gA: 2 × 20 μm, 2 × 50 μm, 2 × 70 μm, Pd/SLB+gA+Ca2+: 2 different devices of 2 × 50 μm and 1 device of 2 × 70 μm. The error bars are the root mean square of the displacement of the data from the average value). Figure 2: Schematics of bioprotonic gA devices. ( a ) Pd contact coated with a SLB. The SLB inhibits the flux of H + from the bulk solution to the Pd/solution interface. ( b ) Pd contact with SLB incorporating gA is semipermeable to H + , with gA channels facilitating the rapid flow of H + to the Pd/solution interface. ( c ) Addition of 1 mM Ca 2+ to the bulk solution, blocks gA and prevents the flow of H + to the Pd/solution interface. ( d ) i H+ versus time plot for V =−200 mV and V =0 mV. Black trace SLB, green trace SLB+gA, blue trace SLB+gA blocked by Ca 2+ . (The data are collected from 3 different devices with different dimensions: Pd / SLB: 3 different devices of 2 × 50 μm, Pd/SLB+gA: 2 × 20 μm, 2 × 50 μm, 2 × 70 μm, Pd/SLB+gA+Ca 2+ : 2 different devices of 2 × 50 μm and 1 device of 2 × 70 μm. The error bars are the root mean square of the displacement of the data from the average value). Full size image In contrast, the bioprotonic device with gA and subjected to V =−200 mV experiences a large i H+ that continually increases to a maximum of i H+ =−4.5 mA cm −2 at t =10 min ( Fig. 2b,d ), because the gA inserted within the SLB create pathways for H + flow. The dependence of i H+ as a function of time will be discussed in the modelling section. Setting V =0 mV after 10 min causes H + to transfer from the PdH x to the solution with a maximum i H+ =0.5 mA cm −2 ( Fig. 2d , green trace). The presence of a large oxidation peak for H + at 50 mV in the I – V sweep confirms that this transfer is indeed occurring ( Supplementary Fig. 4 ). To verify that gA was responsible for H + flow across the SLB, we added 1 mM Ca +2 to block H + transfer across the gA channel ( Fig. 2c ) [25] . Under these conditions, for V =−200 mV we measure i H+ =−0.7 mA cm −2 and subsequently measure i H+ =−0.5 mA cm −2 when setting V =0 mV after 10 min ( Fig. 2d , blue trace). These values of i H+ are comparable to those measured when no gA is incorporated in SLB and are consistent with Ca 2+ blocking gA channels. Alamethicin voltage-gated H + switches To demonstrate that our device architecture can be used to create a voltage-dependent switch that turns the H + flow on and off between bulk solution and isolation layer ( Fig. 3 ), we integrate alamethicin (ALM) into the SLB. Alamethicin is a 20-amino-acids long peptide from the fungus Trichoderma viride . ALM undergoes spontaneous insertion into lipid bilayers and forms a voltage-gated channel when 4-to-6 molecules associate to form an α-helical bundle [54] , [55] , [56] . An asymmetric threshold voltage above ∼ 60 mV induces reorientation of the helices, thereby opening the channel to selective transport of cations, including H + , in the direction of V (ref. 57 ). For V values inferior to this threshold, ALM is closed and there is no H + flow across the membrane in spite of differences in [ H + ], which typically creates a driving force for H + flow ( Fig. 3 ). 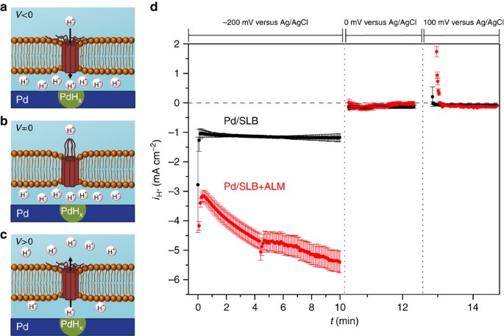Figure 3: Schematics of bioprotonic voltage-gated devices. (a) Pd contact with SLB and ALM. AtV=−200 mV, ALM channels open and H+flows to the Pd/solution interface. (b) PdHxcontact with SLB and ALM remains closed underV=0 mV and there is no H+flow. (c) PdHxcontact coated with SLB and ALM can only oxidize H under a small positive voltage ofV=100 mV which is also required to open ALM channels and allow for flow of H+from the PdHxcontact to bulk solution. (d)iH+versus time plot forV=−200, 0 and 100 mV, SLB black trace and SLB integrating ALM red trace. (The data is collected from 3 different devices with the different dimensions, Pd/SLB: 3 different devices of 2 × 50 μm, Pd/SLB+ALM: 2 × 20 μm, 2 × 40 μm, 2 × 50 μm. The error bars are the root mean square of the displacement of the data from the average value). Figure 3: Schematics of bioprotonic voltage-gated devices. ( a ) Pd contact with SLB and ALM. At V =−200 mV, ALM channels open and H + flows to the Pd/solution interface. ( b ) PdH x contact with SLB and ALM remains closed under V =0 mV and there is no H + flow. ( c ) PdH x contact coated with SLB and ALM can only oxidize H under a small positive voltage of V =100 mV which is also required to open ALM channels and allow for flow of H + from the PdH x contact to bulk solution. ( d ) i H+ versus time plot for V =−200, 0 and 100 mV, SLB black trace and SLB integrating ALM red trace. (The data is collected from 3 different devices with the different dimensions, Pd/SLB: 3 different devices of 2 × 50 μm, Pd/SLB+ALM: 2 × 20 μm, 2 × 40 μm, 2 × 50 μm. The error bars are the root mean square of the displacement of the data from the average value). Full size image Similar to the gA device, we measure i H+ =−5.5 mA cm −2 at V =−200 mV for an ALM integrated bioprotonic device; at V =−200 mV the ALM channel is open, allowing flow of H + ( Fig. 3a,d ). When the voltage is set at V =0 mV, i H+ =0 mA cm −2 . This is because the ALM channel is closed, and no H + flow occurs between IL and B, even after PdH x formation. For V =100 mV, the ALM channel opens and we measure i H+ =1.9 mA cm −2 , indicating that H + flows from the PdH x contact and across the SLB. As a control, we added 40 mM urea to the bulk solution to irreversibly disrupt the ALM channel structure and stop H + flow across the SLB [58] . Under these conditions, we find that i H+ =−1.2 mA cm −2 for V =−200 mV and i H+ =0 mA cm −2 for both V =0 mV and V =100 mV ( Supplementary Fig. 5 ), confirming that ALM is responsible for the bioprotonic device behaviour. Moreover, as is the case with the gA device, the H + oxidation peak at 50 mV dominates the I – V sweep. However, for V >0 mV, i H+ in the ALM device has a rectifying diode-like behaviour ( Supplementary Fig. 6 ). We conclude that the voltage-gated functionality of the ALM channel is maintained on its integration into the device’s SLB. To summarize, the device switches ON when ALM voltage-gated channels are open, allowing H + flow across the membrane and in the direction of V . The device is OFF when V =0 mV, a voltage below the threshold value needed for ALM opening. Thus, an ALM device can be used to modulate H + flow and [ H + ] between IL and B, much like cells control [ H + ] differences between cytosol and extracellular space. A model for H + transfer across gA and ALM channels To better understand the dynamics of H + flow in our biotic–abiotic devices, we modelled H + transport characteristics using the Nernst–Plank equation to fit our device current density data, i H+ ( Fig. 4 ). To this end, we divide the device into four distinct layers: the bulk solution (B); a Supported Lipid Bilayer membrane (SLB) with variable permeability ( P SLB ) that encompasses the SLB with integrated gA or ALM; the isolation layer (IL); and the Pd/PdH x contact ( Fig. 4a ). When a negative voltage −V is applied to the Pd contact, H + flow from B across the SLB and into the IL. We quantify this transport as the H + current density across membrane, j H+ . A portion of the H + from j H+ contribute to an increase in [ H + ] in the IL, [ H + ] IL , while the remaining H + are reduced to H at the Pd contact and form PdH x . We assume that i H+ measured between the Pd contact and the Ag/AgCl electrode arises entirely from electrons participating in H + oxidation (positive i H+ ) or reduction processes (negative i H+ ), and we quantify it as current density, i H+ . 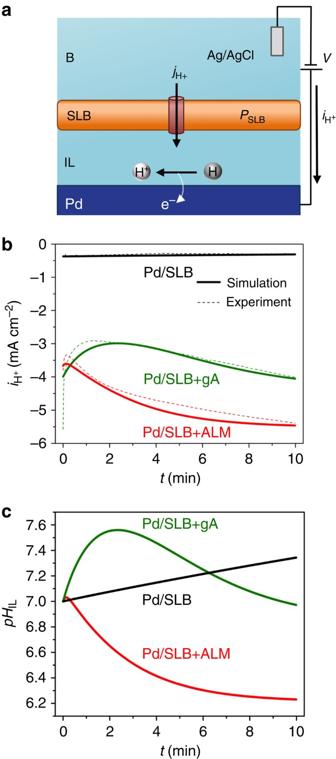Figure 4: Analytical description of channel permeability. (a) Schematic of membrane modelling parameters. (B, bulk solution; SLB, Supported Lipid Bilayer membrane; IL, isolation layer;PSLB, SLB permeability; [H+]IL, H+concentration in isolation layer;jH+, H+flux across the membrane;iH+, H+redox current density;V=−200 mV;jH+andiH+are computed with equations 2 and 3, respectively. A rise in [H+]ILincreases the d[H+] between Ag/AgCl electrode and Pd contact for H+reduction, according to the Nernst equation (equation 4). (b) Iterative simulation ofiH+at the Pd/solution interface for SLB (black trace), SLB incorporating gA (green trace), and SLB incorporating ALM (red trace) bioprotonic device. A combination of GHK and Tafel equations was used to describe the behaviours of membrane and Pd contact. (c) Change inpHILusing the parameters from the simulation. Figure 4: Analytical description of channel permeability. ( a ) Schematic of membrane modelling parameters. (B, bulk solution; SLB, Supported Lipid Bilayer membrane; IL, isolation layer; P SLB , SLB permeability; [ H + ] IL , H + concentration in isolation layer; j H+ , H + flux across the membrane; i H+ , H + redox current density; V =−200 mV; j H+ and i H+ are computed with equations 2 and 3, respectively. A rise in [ H + ] IL increases the d[ H + ] between Ag/AgCl electrode and Pd contact for H + reduction, according to the Nernst equation (equation 4). ( b ) Iterative simulation of i H+ at the Pd/solution interface for SLB (black trace), SLB incorporating gA (green trace), and SLB incorporating ALM (red trace) bioprotonic device. A combination of GHK and Tafel equations was used to describe the behaviours of membrane and Pd contact. ( c ) Change in pH IL using the parameters from the simulation. Full size image From conservation of mass (equation 1) [59] where, e is elementary charge=1.6 × 10 −19 C, and d[ H + ] IL is the incremental change in molar concentration of H + in the IL in moles m −3 . j H+ is obtained by inserting the Goldman–Hodgkin–Katz (GHK) solution [60] into the Nernst–Planck equation (equation 2) [59] : where P SLB is the permeability of H + through the SLB, F is Faraday’s constant, f is F/RT, or 38.66 V −1 , V m is the potential difference across the membrane and [ H + ] B is the H + concentration in the bulk layer in moles m −3 (10 −4 mol m −3 ). We set V m = V and assume that the potential drop across B is negligible relative to the potential drop across the membrane. When no gA or ALM channels are present, the resistance of the SLB, R SLB ≈GΩ ( Figs 2 and 3 ), is six orders of magnitude higher than the resistance of B ( R B =0.6 kΩ). We derive i H+ using a modified version of the Tafel equation [61] (equation 3): where i 0 is the Pd exchange current density (a constant describing forward and reverse i H+ at the Pd/solution interface when they are equal to each other and the net i H+ is 0 mA cm −2 ), α is the transfer coefficient, V 0 is the redox potential between Pd and Ag/AgCl (−0.22233 V), and V N is the Nernstian potential created by the change in [ H + ] across the SLB. V N is derived from (equation 4): We assume that [ H + ] B remains constant and calculate the change in [ H + ] IL from the change of pH in the IL, d pH IL , assuming a buffering capacity for the solution, β ( Supplementary Note 2 ) [62] : where D IL is the thickness of the isolation layer. The resulting d[ H + ] IL is (ref. 59 ): To fit i H+ to the experimental data, we programed an iterative solution to the above model using the membrane permeability, P M , as a fitting parameter. For V =−200 mV and D IL =0.5 nm the model fits the experimental data well using membrane permeabilities of P SLB =0.006 s −1 (unmodified SLB), P SLB+gA =0.58 s −1 (SLB with integrated gA) and P SLB+ALM =0.74 s −1 (SLB with integrated ALM). Consistent with our expectation, insertion of either gA or ALM into the SLB increases membrane permeabilities by three orders of magnitude. We did not control or accurately measure the density of the channels and these permeabilities are characteristic of the device and do not represent the absolute conductivities of individual gA or ALM. We next calculate the change in pH IL using the above permeabilities ( Fig. 4c ). Qualitatively, if the rate at which H + are reduced at the Pd contact is higher than the rate at which H + permeate the membrane (| i H+ |>| j H+ |), pH IL will increase with respect to the pH B . Considering protochemical potential differences among B, IL and the Pd/PdH x contact, an acidic pH IL will favour transfer of H + from the IL into Pd (| i H+ |>| j H+ |), while a basic pH IL will favour transfer of H + from B to the IL through the gA and ALM channels. For a naked SLB, our model predicts that some H + reduction will occur at the Pd surface. Very few H + leak through the membrane and pH IL increases slowly ( Fig. 4c , black trace). For an SLB integrating gA, the model predicts an initial increase in pH IL followed by a progressive decrease as more H + flow through the gA channel over time. These results can be rationalized as follows: at the initial pH IL =7, reduction at the Pd contact interface (| i H+ |) is favoured with respect to flow through gA channels (| j H+ |) because pH B = pH IL and the only driving force for flow along the gA channel is V . As pH IL increases, | j H+ | increases and | i H+ | decreases ( Fig. 4b ) due to the [ H + ] difference between B and IL driving H + flow across gA. In the case of an SLB integrating ALM, the dynamics for i H+ and pH IL are essentially the same as for gA but with a shorter time constant and a lower pH IL plateau value. This is likely due to the fact that P ALM > P gA : the higher membrane permeability of ALM SLBs favours H + transfer (| j H+ |) over H + reduction at the Pd/PdH x interface (| i H+ |). In summary, the model developed with our bioprotonic devices provides information on the H + permeability of biomimetic membranes. It should prove valuable to characterize the transport behaviour of other ion channels or H + pumps in biotic–abiotic devices. In this communication, we demonstrate a biotic–abiotic bioprotonic device with proton (H + ) conducting Pd/PdH x contacts that measures and controls the flow of H + across a lipid bilayer with the ion channels gramicidin A (gA) and alamethicin (ALM). We use gA to increase membrane permeability and control the H + flow across the lipid bilayer with a voltage applied on the Pd/PdH x contact. We also demonstrate bidirectional voltage gated switching of the H + flow across the SLB with ALM. Finally, we model H + transport in this system using the Goldman solution and the Nernst equation and use the model to derive the permeability parameters of the lipid bilayer with integrated gA and ALM ion channels and to predict change in pH of the solution at the lipid bilayer/Pd contact interface. Our results indicate that ion channels increase SLB permeability by three orders of magnitude. This is the first time that H + conducting channels have been integrated with Pd/PdH x H + -conducting contacts and that the H + current flowing through these channels has been directly measured and controlled. Future integration of more complex proteins may require Pd contact functionalization with a self-assembled monolayer [63] or cushioning lipopolymer [64] , [65] , [66] to passivate the Pd surface and overcome protein denaturation [66] . To this end, we demonstrate that passivation of the Pd contact with self-assembled 3-aminopropyl-triethoxy-silane [63] retains gramicidin A device functionality ( Supplementary Figs 7–9 ). On the other hand, passivating the Pd contact with poly (ethylene glycol) [67] , [68] insulates the Pd surface and hampers H + transfer at the Pd contact solution interface. Alternatively, larger proteins such as H. turkmenica detarhodhopsin can be engineered to bind to the Pd contact surface without experiencing denaturation by making use of fused Pd-binding peptides [69] . This work opens the door to integrating more complex active H + channels at the Pd contact interface to produce biotic–abiotic devices with increased functionality. Materials 1,2-dioleoyl-sn-glycerol-3-phosphocholine (DOPC; Sigma-Aldrich), Bacillus brevis Gramicidin A (90% purity; BioChemika), Trichoderma viride Alamethicin (90% purity; Sigma-Aldrich) were used as received. The heterofunctional PEG, 1,2-distearoyl-snglycero-3-phosphoethanolamine-N-poly (ethylene glycol)-2000-N- (3-(2-(pyridyldithio) propionate) (DSPE-PEG-PDP) and lipids, L-R-phosphatidylcholine from egg (egg-PC), were purchased from Avanti Polar Lipids (Alabaster, AL). 3-aminopropyl-triethoxy-silane was purchased from, Sigma-Aldrich. Potassium ferrocyanide (K 4 (Fe(CN) 6 ), 99.9% purity) K 2 HPO 4 , KH 2 PO 4 , KCl, HCl and KOH (all with 99.9% purity) were purchased from Sigma-Aldrich. K-PBS buffer consisted of 100 mM KCl in 5 mM potassium phosphate (K 2 HPO 4 /KH 2 PO 4 at a molar ratio of 3:2), pH=7.0. Buffer solutions were prepared with degassed deionized water (Millipore) and the pH was adjusted to 7.0 with HCl or KOH if necessary. The reference and counter electrode (1-mm diameter 3 M KCl Ag/AgCl) was from Warner Instruments. Silicon wafers (100), 4-in. diameter were acquired from International Wafer Service. Ethanol, (200 proof), acetone and chloroform had 99.9% purity. Device fabrication and characterization Bioprotonic devices were fabricated with conventional soft- and photo-lithography on a 100 nm thick layer of silicon dioxide. Each device has a microfluidic SU-8 channel of 4 μm thick. The Pd contacts have varied contact area of 10 μm 2 (2 × 5 μm), 20 μm 2 (2 × 10 μm), 40 μm 2 (2 × 20 μm), 80 μm 2 (2 × 40 μm), 100 μm 2 (2 × 50 μm), 120 μm 2 (2 × 60 μm), 140 μm 2 (2 × 70 μm), 160 μm 2 (2 × 80 μm), 180 μm 2 (2 × 90 μm) and 200 μm 2 (2 × 100 μm) with a thickness of 50 nm. Pd is deposited on top of 5 nm Cr adhesion layer. Each device has an electrical probe pad out of the microfluidic channel that provides the electrical contact. The microfluidic channel confines the flow of liquid to the top of the Pd contact, while a polydimethylsiloxane well on top of the channel provides space to insert the counter electrode ( Supplementary Fig. 1 ). SLB formation and characterization DOPC vesicles ( d avg =100±23 nm, n =3) were prepared by tip sonication of a solution of 0.5 mg ml −1 DOPC, in K-PBS buffer solution (pH=7.0). Dynamic light scattering was used to characterize vesicle size. Before deposition, the Pd surface was hydrophilized by oxygen plasma [70] . The vesicle solution was dispensed in the microfluidic channel and the device was gently agitated for 12 h at 100% relative humidity to ensure vesicle fusion, followed by rinsing with K-PBS buffer solution to wash away unfused DOPC vesicles. The resulting bilayers were characterized by AFM, with rupture depth measurements showing a thickness of ca. 4.8±0.7 nm ( Supplementary Fig. 2 and Supplementary Note 1 ) [46] . Home-built systems were used to conduct cyclic voltammetry experiments in the presence of a redox probe and I – V measurements in the presence of buffer solution. Throughout this process, the pH was monitored using a calibrated pH metre. Ion channel incorporation into supported lipid bilayers Gramicidin A (5 mg ml −1 ) in 200-proof ethanol was mixed with DOPC in chloroform followed by solvent evaporation with N 2 the rehydration with aqueous buffer solution. DOPC/gramicidin vesicles at a molar ratio of 200:1 were formed by tip sonication and vesicle size determined by dynamic light scattering ( d avg =105±26 nm, n =3). These vesicles were then fused onto Pd microfluidic devices. ALM was incorporated into bilayers by incubating 5 mg ml −1 solution of ALM peptide for 30 min on freshly deposited Pd-bilayer structures followed by rinsing with K-PBS buffer solution. Electrical measurements All electrical measurements were performed using a Signatone S probe station with a custom built environmental chamber. The probe station was connected to an Agilent 4155C semiconductor parameter analyser. Simulations Iterative simulations were executed in the MATLAB software package. Pd contact Tafel parameters i 0 and α were measured with low-voltage I – V sweeps at a scan rate of 5 mV s −1 ( Supplementary Fig. 10 ). The permeability of the three membranes were estimated using a composite model of the permeability of individual cationic channels and the permeability of the DOPC matrix, normalized to their respective occupied area. The length of the isolation layer (ca. 1 nm) was estimated using AFM force versus displacement measurements. Code availability MATLAB code for simulations is available at https://dx.doi.org/10.6084/m9.figshare.3509846.v1 . Data availability The data that support the findings of this study are available from the corresponding author on request. How to cite this article: Hemmatian, Z. et al . Electronic control of H + current in a bioprotonic device with Gramicidin A and Alamethicin. Nat. Commun. 7, 12981 doi: 10.1038/ncomms12981 (2016).